Structural and molecular insights into the mechanism of action of human angiogenin-ALS variants in neurons Mutations in angiogenin ( ANG ), a member of the ribonuclease A superfamily, are associated with amyotrophic lateral sclerosis (ALS; sporadic and familial) and Parkinson's disease. We have previously shown that ANG is expressed in neurons during neuro-ectodermal differentiation, and that it has both neurotrophic and neuroprotective functions. Here we report the atomic resolution structure of native ANG and 11 ANG-ALS variants. We correlate the structural changes to the effects on neuronal survival and the ability to induce stress granules in neuronal cell lines. ANG-ALS variants that affect the structure of the catalytic site and either decrease or increase the RNase activity affect neuronal survival. Neuronal cell lines expressing the ANG-ALS variants also lack the ability to form stress granules. Our structure–function studies on these ANG-ALS variants are the first to provide insights into the cellular and molecular mechanisms underlying their role in ALS. Amyotrophic lateral sclerosis (ALS) is a late onset neurodegenerative disorder in which upper and lower motor neurons (MNs) are selectively killed leading to paralysis with extremely poor prognosis. Most known cases of ALS are sporadic, but ~10% are familial and until a decade ago mutations in the SOD1 (the gene encoding Cu/Zn superoxide dismutase) was one of the main known causes of ALS. Since then mutations in other genes such as ALSIN , VAPB , SETX , OPTN , FUS/TLS , TARDP , UBQLN2, FIG4, C9ORF72 and VEGF have also been shown to be associated with ALS [1] , [2] , [3] , [4] . Mutations in angiogenin ( ANG ) are implicated in ALS, both familial and sporadic [5] , [6] . Several other studies worldwide have also identified ANG mutations in ALS patients [7] , [8] , [9] , [10] , [11] , [12] , [13] , [14] , [15] , [16] , [17] . 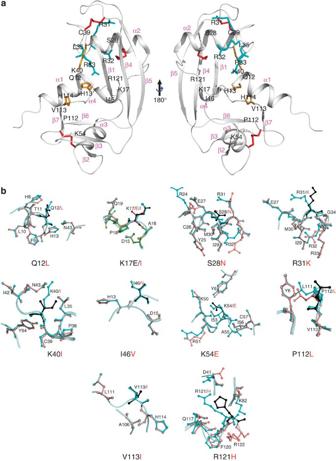Figure 1: 3D structure of hANG and the comparison of hANG-ALS variant structures at the mutation sites. (a) High-resolution structure of native hANG. The active site residues (orange) and the nuclear localization sequence (cyan) are shown. Labelled in black are the positions of hANG-ALS variants in the ANG structure. The disulphide bridges are shown as red sticks. Labelled in purple are the secondary structure elements of hANG. Figure was created using the programme PyMOL (http://www.delanoscientific.com). (b) Structural comparison of hANG and ALS-associated variants. Superposition of native hANG (in cyan) and hANG-ALS (in salmon except for the mutant in black) variants. Residues that exhibit hydrogen-bonding interactions with the hANG-ALS residues both in native hANG and mutant structures are also shown. K17/I is shown in firebrick colour, whereas the hydrogen-bonding residues are shown in pea colour. More recently a large multi-site study reported the association of mutations in ANG with ALS as well as Parkinson's disease (PD) [8] , [18] ( Table 1 ). ANG has also been shown to have a neuroprotective effect in a mouse model of PD [19] . Many of the proteins implicated in ALS, such as ANG, TDP-43 and FUS, belong to the RNA processing and metabolism pathways. There is growing evidence that MN degeneration in ALS may be linked to errors in multiple steps of RNA metabolism or processing [20] , [21] , [22] . Table 1 Reported hANG mutations implicated in ALS. Full size table Human angiogenin (hANG) [23] , [24] , [25] is an angiogenic molecule that induces neovascularization [26] . It is a monomeric protein of 14.1 kDa that belongs to the pancreatic ribonuclease A (RNase A) superfamily [27] . ANG has the same catalytic properties as RNase A: it cleaves preferentially on the 3′ side of pyrimidine and follows a transphosphorylation/hydrolysis mechanism [28] , [29] . The crystal structure of hANG has revealed that it has a RNase A fold and the catalytic triad (residues H13, K40 and H114) is conserved ( Fig. 1 ) [30] . The enzymatic activity of ANG is several orders of magnitude lower than that of RNase A towards conventional RNase substrates [29] . The weak ribonucleolytic activity and the translocation of ANG to the nucleus [31] are essential to the angiogenic process [28] , [32] . Figure 1: 3D structure of hANG and the comparison of hANG-ALS variant structures at the mutation sites. ( a ) High-resolution structure of native hANG. The active site residues (orange) and the nuclear localization sequence (cyan) are shown. Labelled in black are the positions of hANG-ALS variants in the ANG structure. The disulphide bridges are shown as red sticks. Labelled in purple are the secondary structure elements of hANG. Figure was created using the programme PyMOL ( http://www.delanoscientific.com ). ( b ) Structural comparison of hANG and ALS-associated variants. Superposition of native hANG (in cyan) and hANG-ALS (in salmon except for the mutant in black) variants. Residues that exhibit hydrogen-bonding interactions with the hANG-ALS residues both in native hANG and mutant structures are also shown. K17/I is shown in firebrick colour, whereas the hydrogen-bonding residues are shown in pea colour. Full size image hANG is expressed strongly in the human spinal cord [16] and in the developing nervous system of the mouse as well as during neuronal differentiation of pluripotent stem cells, suggesting a role for this protein in the nervous system [33] . It has neurotrophic and neuroprotective function [33] , [34] in the central nervous system and the loss of this activity may be a causal mechanism for ALS [34] , [35] , [36] , [37] . hANG binds to DNA and stimulates transcription and/or processing of pro-ribosomal RNA [38] , [39] , thereby participating in the increased production of ribosomes, which may be important for the normal physiological function of MNs [16] , [24] . Recent findings show that ANG is a stress-activated RNase that cleaves tRNA. These fragments can inhibit translation initiation and is key to stress response and cell survival [40] , [41] , [42] , [43] . In this report, we decipher the molecular interactions of 11 hANG-ALS variants (elucidated by X-ray crystallography) and compare them with the newly determined high-resolution structure of the native protein. The structural information is correlated with their effects on hANG uptake by neurons, neuronal survival and stress granule (SG) assembly in neuronal cell lines. Our findings provide insights into the molecular interactions that are altered in the hANG-ALS variants leading to functional effects. Overview We have determined the crystal structures of native ANG (1. 04 Å) and 11 ANG-ALS variants ( Table 1 , in the resolution range 2.97–1.96 Å, Supplementary Table S1 ). The high-resolution structure of native ANG enabled us to look closely at the perturbations in the vicinity of the ALS mutations. Atomic resolution structure of hANG The active site of ANG molecule consists of several sub-sites: a P 1 substrate-binding site involved in phosphodiester bond cleavage; a B 1 site for binding the pyrimidine whose ribose donates its 3′ oxygen to the scissile bond; a B 2 site that preferentially binds a purine ring on the opposite side of the scissile bond; and additional sites for peripheral bases and phosphates [30] . In the atomic resolution structure of native ANG ( Supplementary Table S1 , Fig. 1 ), several residues (T7, P18, Q19, G20, R21, S28, R31, S37, K40, D41, S52, P64, S72, K73, T97 and A98) were found to have multiple side-chain conformations compared with the previously reported lower-resolution structure [30] . Conformational flexibility was also observed in the region spanning residues 16–20, which has implications for substrate binding. Dual conformation was also observed for the NZ atom of K40, which is a part of the catalytic triad. In one of the conformations, this NZ atom makes a strong hydrogen bond interaction with the main chain carbonyl oxygen atom of I42 and OD1 of N43. 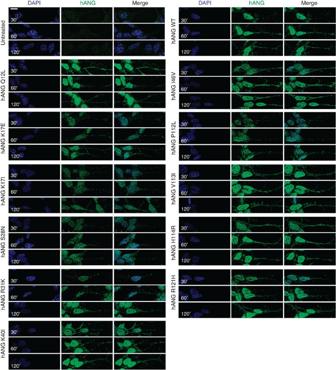Figure 2: Uptake and localization of WT hANG and hANG-ALS variants in SY5Y cells. SY5Y neuronal cells were incubated with the hANG variants at 200 ng ml−1for 30, 60 and 120 min as described in Methods. Cells were fixed in ice-cold methanol for 15 min immunostained using the 26-2F mAb to hANG and visualized using an Alexa 488-conjugated anti-mouse antibody. Nuclei were counterstained with DAPI. Negligible staining is seen in untreated cells. WT hANG is seen in the nucleus, cytoplasm and neurites at 120 min. R31K and S28N variants undergo nuclear translocation by 120 min. Variants in which the catalytic activity is affected also undergo nuclear translocation. The Q12L and the K40I variants are present at high levels in the nucleus as large speckles by 30 min and staining on the cell membrane is very strong. At 120 min, the K40I variant is mostly nuclear with strong staining on the cell membrane and in the cytoplasm, the Q12L mutant on the other hand is present at low levels in the nucleus but is strongly present in the neurites and the cell membrane. The uptake and the intracellular distribution of V113I variant is similar to the K40I at 30 min but at 120 min is weakly present in the cytoplasm and neurites. The H114R variant is present very strongly on the cell membrane, nucleus, cytoplasm and neurites at 30 min, but by 120 min there is still strong nuclear staining with fine vesicular staining on the cell membrane but weak staining in the cytoplasm and neurites. The R121H variant localizes to the nucleus with negligible staining in the cytoplasm and cell membrane at 30 min, but at 60 min there is diffuse cytoplasmic staining and weak staining in the nucleus, neurites and the cell membrane. However, by 120 min there is strong staining in the nucleus, neurites and cell membrane. The K17I variant is undetectable in the nucleus at 30 and 60 min and is weakly present at 120 min. The K17E variant is seen in the nucleus at 30 and 120 min, and there is staining in the nucleus and neurites. Scale bar, 25 μm. In the alternate conformation, the NZ atom of K40 interacts with the OE1 atom of Q12 and NE2 of H13 through a water-mediated hydrogen bond interaction, and a direct hydrogen bond with the OD1 atom of N43 ( Table 2 , Supplementary Fig. S1a ). All these interactions are important for catalysis. Residue R31, which is part of the nuclear localization sequence (NLS) 31 R-R-R-G-L 35 , also exhibits dual conformation. The OG atom of S28 was also found to display dual conformation. In the most predominant conformation (occupancy 0.76), the OG atom interacts with NH1/2 atom of R32 through a strong hydrogen bond (2.84 Å). Residue S28 appears to hold R32 (which is part of the NLS) in position ( Table 2 , Supplementary Fig. S1b ). Table 2 Hydrogen bond and van der Waals contact residues in hANG and hANG-ALS variants. 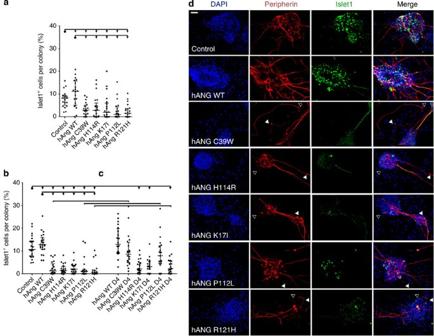Figure 3: Effects of WT hANG and hANG-ALS variants on post-mitotic motor neuron (MN) number and morphology. P19 cells were induced to differentiate to MNs by plating on PA6 feeder cells in the presence of RA as described inSupplementary Methods. Cells were differentiated in the presence or absence of hANG and hANG-ALS variant proteins from days 0 to 5 (a) and day 6 (b), or from days 4 to 6 only (c). Immunostaining for Islet 1 and Peripherin was used to determine the number of MNs per colony, whereas the total number of nuclei in a colony was found by DAPI staining, as described inSupplementary Information. Data were collected from two independent experiments (n≥10 colonies for each experiment). Median bars with interquartile range. Ball and arrow bars show where multiple conditions are significantly different from a single condition, whereas solid bars show significant differences between two conditions (P0.05, Logetransformed data compared by analysis of variance with Tukey'spost hoc). (d) Cells fixed on day 6 and stained for Peripherin (red) and Islet 1 (green) and counterstained with DAPI (blue). Cells were differentiated either in the absence of ANG (control) or in the presence of ANG WT, C39W, H114R, K17I, P112L or R121H variants. Filled arrows indicate kinked neurites. Hollow arrows indicate fragmented neurites. Scale bars, 50 μm. Full size table Key features of hANG-ALS variant crystal structures Biochemical characterization of hANG-ALS variants ( Table 1 ) showed that only the R121H variant has an elevated level of RNase activity (that is, activity towards tRNA; ~55% more) compared with native ANG, whereas others show low ribonucleolytic activity in the range of 0.7–90% ( Table 3 , Supplementary Fig. S2a ). Circular dichroism spectroscopy showed that all these variants of hANG retain the overall fold of the native structure in solution ( Supplementary Fig. S2b ). Table 3 Structural deviation and solvent accessibility changes caused by hANG-ALS variants. Full size table We have determined the crystal structures of hANG variants—Q12L, K17E, K17I, S28N, R31K, K40I, I46V, K54E, P112L, V113I and R121H ( Supplementary Table S1 ). In several structures, significant local changes in conformation/environment were observed ( Fig. 1b , Supplementary Fig. S8 , Tables 2 , 3 ). Key features of hANG-ALS variant structures Q12 in ANG is part of the P 1 substrate-binding sub-site and a conserved residue across different species ( Supplementary Table S2 ). In the variant structure ( Fig. 1b ), mutation of Q12 to Leu (polar to hydrophobic) reduces the solvent accessibility ( Table 3 ), affects T44 through van der Waals interactions and a loss of H-bond potency with L10. In the native structure, T44 interacts with Q117 (part of the pyrimidine recognition site) and T80, a substrate-binding residue ( Table 2 ). Hence, the significant loss of RNase activity in the variant appears to be due to the deleterious effect of the hydrophobic Leu residue in the active site of ANG. Both the hANG-ALS variants K17E/I exhibit significant decrease (5-8 fold, respectively) in ribonucleolytic activity of the enzyme. It has been shown previously that residues 8–22 are important for the action of hANG in intact ribosomes and mutations in this region lead to a marked decrease in inhibition of cell-free protein synthesis [44] , [45] . Comparison of ANGs from different species shows that residue K17 is generally conserved and the basic charge appears to be important at this position ( Supplementary Table S2 ). In the X-ray structures of hANG (native) and the K17E/I variants ( Fig. 1b ), the loop region 16–20 (which contains the P18 residue) exhibits a high degree of flexibility and is possibly involved in substrate binding as part of a peripheral recognition site for rRNA. It is also in close proximity to the NLS region ( 31 R-R-R-G-L 35 ). The K17E variant retains the full complement of van der Waals interactions similar to the native hANG. However, the K17I variant has lost its H-bond interaction with D15, which is compensated by an H-bond interaction with Q19 ( Table 2 ). Wu et al . [16] reported that the variant S28N had negligible angiogenic activity and diminished RNase activity as compared with native ANG. However, we found that S28N variant retains ~20% of ribonucleolytic activity ( Supplementary Fig. S2a ). The Ser residue is conserved in ANGs from most species ( Supplementary Table S2 ). In the native structure, S28 is located in a helix near the active site. At the tip of this helix is the key catalytic lysine (K40) presented by a small loop. Furthermore, this residue is close to the flexible loop region 16–20 of hANG (as described above). Thus, it is expected that any significant change in this residue will affect the structure of the flexible loop region. In the variant structure, there is an increase in solvent accessibility ( Table 3 ). In addition, local conformational changes involving the NLS 31 R-R-R-G-L 35 were observed in the variant structure ( Fig. 1b , Supplementary Fig. S1b , Table 2 ), in particular, the R32 side chain adopts a different conformation because of the loss of a key H-bond between S28 and R32 present in the native hANG structure. Amino-acid residue R31 is part of the NLS of hANG [31] . It has previously been shown that the variant R31K does not affect the biological and/or ribonucleolytic activity of hANG. It is also known that in several species Arg is replaced by Lys ( Supplementary Table S2 ). In the crystal structure of the variant ( Fig. 1b ), the mutated residue Lys is less solvent accessible ( Table 3 ) and does not make H-bond interaction with E27 ( Table 2 ), which may result in slight loss of activity (~8%) but will have little influence on the nuclear translocation. The ANG-ALS variant C39W has very low ribonucleolytic activity ( Supplementary Fig. S2a ). This mutation eliminates a disulphide bridge with C92 that is conserved throughout the pancreatic RNase A superfamily ( Supplementary Table S2 ). It is known that removal of the corresponding disulphide bond in RNase A decreases enzymatic activity by 11-fold (Ala mutations) or 20-fold (Ser mutations) similar to the present findings for C39W variant [46] . In addition, our molecular modelling study predicts that the new Trp residue in C39W might cause significant perturbations that have an effect on catalytic activity beyond that due to simple loss of the stabilizing disulphide. Although the mutation does not appear to have direct involvement in catalysis it does affect the stability of the enzyme [46] . The recombinant expression of this variant protein has been straight forward, but crystallization trials so far have failed to yield crystals suitable for structural study. Lys40 is a key residue at the catalytic centre (P 1 sub-site) [30] of ANG and the substitution by the Ile residue (less solvent accessible, Table 3 ) abolishes the catalytic and biologic activity of the protein [46] . In the crystal structure of the ALS variant K40I, several key interactions of K40 (with residues Q12, C39, N43 and T44, which are integral part of the catalytic site) known to be important for the stabilization of the transition state during RNA cleavage are lost ( Table 2 , Fig. 1b ). This has extensive repercussions throughout the active site region. Ile46 is a conserved residue among ANG sequences (except in rabbit where it is replaced by Val, Supplementary Table S2 ) and the mutation to Val results in tenfold decrease in RNase activity and thermal stability [46] . In both native and the variant structures ( Tables 2 , 3 ), this residue is located in a hydrophobic core of the molecule. Even though no major changes in the H-bond interactions were observed, the variant appears to have substantially fewer number of van der Waals contacts 35 versus 49 (in the native) involving residues (H13, Y14, D15) from the amino-terminal helix that are part of the catalytic site ( Fig. 1a,b ). Lys54 is conserved in most species ( Supplementary Table S2 ). This residue does not participate or belong to any of the known catalytic sub-sites of the enzyme [30] . The variant K54E retains 80% of RNase activity. In the variant structure, this residue is exposed on the surface of the molecule ( Table 3 ), but this change alone is not sufficient to explain the loss of 20% RNase activity. It is likely that the basic nature of the mutated residue in the variant will have an influence on the catalytic activity through a new interaction with residue Y6 and a minor rearrangement of the N-terminal helix involving the catalytically important residue H13 ( Fig. 1b , Table 2 ). The residues Pro112, Val113 and His114 are conserved among RNase A superfamily of enzymes and form part of the catalytic apparatus ( Table 2 ). Substitution at these positions results in loss of function of ANG. In case of the V113I variant, a nonpolar residue Val is substituted by Ile, which is also nonpolar. However, the additional methyl group from Ile ( Fig. 1b ; at the catalytic sub-site) may lead to steric conflicts for substrate binding, which could account for loss of ~25 % RNase activity. Similar to the report by Wu et al . [16] , we also find that the P112L mutation results in ~70 % loss of RNase activity of ANG. Proline has a unique cyclical structure compared with the other 19 commonly occurring amino acids and normally provides conformational stability in three-dimensional (3D) structures. In the native ANG structure, P112 is located near the catalytic sub-site and mutation to a Leu residue in the variant resulted in significant perturbations ( Fig. 1b ) at the carboxy-terminal region ( Table 2 ) that could account for low catalytic efficiency. The Leu substitution at position 112 also affects the NLS. H114 is a key catalytic site residue in ANG [32] and mutation of this residue to Ala or Asn would result in a 10,000- or 3,300-fold reduction in RNase activity, respectively, as compared with the native protein. Our studies show that the RNase activity of the H114R variant is abrogated ( Supplementary Fig. 2a , Table 3 ). We do not as yet have the structure of the H114R variant. However, we speculate that the longer side chain of Arg (compared with the imidazole ring of the catalytic His residue; Fig. 1a ) would disrupt the catalytic site thereby affecting the cleavage of phosphodiester bond, which could account for the major loss of RNase activity. An important structural feature of ANG compared with RNase A is that a part of the active site (that is, part of the C-terminal region of the molecule spatially analogous to that for pyrimidine binding in RNase A) is 'obstructed' by residue Q117 (ref. 30 ). Movement of Q117 and adjacent residues is required for substrate binding to ANG, hence, constitutes a key part of its mechanism of action [47] . Indeed, previous studies on the mutation of D116 (ref. 48 ) and/or Q117 of ANG to Ala/Gly showed increased RNase activity by 11- to 30-fold by the variants towards their substrates [47] . In addition, mutational studies on C-terminal segment have shown that shorter side-chain residues or deletion of residues exhibit enhanced ribonucleolytic activity [49] . Consistent with this view, the Q117G, D116H and I119A/F120A variants are 4- to 30-fold more active than hANG. In addition, crystal structures for these variants have shown that in all three cases, the C-terminal segment remains obstructive, demonstrating that none of the residues that have been replaced is essential for maintaining the closed conformation [50] . The Q117G structure showed no changes other than the loss of the side chain of residue 117, whereas those of the D116H and I119A/F120A revealed C-terminal perturbations beyond the replacement site, suggesting that the native closed conformation has been destabilized [50] , [51] . In the I119A/F120A variant structure, the segment containing residues 117–123 is highly mobile and all of the interactions thought to position Q117 are weakened or lost; the space occupied by F120 in ANG was partially filled by R101, which has moved several angstroms [52] . In the 3D structure of native ANG, R121 forms part of a peripheral sub-site for binding polynucleotide substrates at the C-terminal region. The ALS-associated variant R121H has significantly higher RNase activity as compared with native hANG. In the crystal structure of R121H variant ( Fig. 1b ), the smaller side chain of histidine appears to provide a 'spatial opening' ( Table 2 ; upon binding of the substrate) of the obstructive pyrimidine-binding site thereby allowing better access for substrate binding, which would explain the enhanced RNase activity. Recently, four new hANG-ALS variants—T80S [8] , F100I [8] , V103I [7] and R121C [9] —were reported ( Table 1 ). Detailed biochemical and structural characterization of these variants are currently underway. The predicted likely structural features are described in Supplementary Note 1 . Uptake of hANG-ALS variants by SY5Y cells Wild-type (WT) hANG when added to cells in culture is taken up and translocated to the nucleus [31] . To investigate whether the ALS-associated mutations affect the uptake and translocation of ANG to the nucleus, we exposed the human neuronal cell line SY5Y to hANG and hANG-ALS variants (for which we have determined the 3D structure) and detected uptake by staining with the 26-2F monoclonal antibody to hANG ( Fig. 2 ). The untreated control cells show low-level staining for hANG in the cytoplasm. The antibody 26-2F is specific to the WT human ANG and will recognize the endogeneous hANG produced by the SY5Y cells. SY5Y cells incubated with WT hANG for 30 min exhibit strong staining in the nucleus, some staining in vesicles in the cytoplasm and in the neurites. The staining intensity increases at 60 min and by 120 min, the nucleus, neurites and the cell membrane all exhibit strong staining ( Fig. 2 ). Figure 2: Uptake and localization of WT hANG and hANG-ALS variants in SY5Y cells. SY5Y neuronal cells were incubated with the hANG variants at 200 ng ml −1 for 30, 60 and 120 min as described in Methods. Cells were fixed in ice-cold methanol for 15 min immunostained using the 26-2F mAb to hANG and visualized using an Alexa 488-conjugated anti-mouse antibody. Nuclei were counterstained with DAPI. Negligible staining is seen in untreated cells. WT hANG is seen in the nucleus, cytoplasm and neurites at 120 min. R31K and S28N variants undergo nuclear translocation by 120 min. Variants in which the catalytic activity is affected also undergo nuclear translocation. The Q12L and the K40I variants are present at high levels in the nucleus as large speckles by 30 min and staining on the cell membrane is very strong. At 120 min, the K40I variant is mostly nuclear with strong staining on the cell membrane and in the cytoplasm, the Q12L mutant on the other hand is present at low levels in the nucleus but is strongly present in the neurites and the cell membrane. The uptake and the intracellular distribution of V113I variant is similar to the K40I at 30 min but at 120 min is weakly present in the cytoplasm and neurites. The H114R variant is present very strongly on the cell membrane, nucleus, cytoplasm and neurites at 30 min, but by 120 min there is still strong nuclear staining with fine vesicular staining on the cell membrane but weak staining in the cytoplasm and neurites. The R121H variant localizes to the nucleus with negligible staining in the cytoplasm and cell membrane at 30 min, but at 60 min there is diffuse cytoplasmic staining and weak staining in the nucleus, neurites and the cell membrane. However, by 120 min there is strong staining in the nucleus, neurites and cell membrane. The K17I variant is undetectable in the nucleus at 30 and 60 min and is weakly present at 120 min. The K17E variant is seen in the nucleus at 30 and 120 min, and there is staining in the nucleus and neurites. Scale bar, 25 μm. Full size image The hANG-ALS variants show differences in the kinetics of uptake as well as in the intracellular distribution. The R31K variant, which affects the NLS, and the S28N variant, which is in the vicinity of the NLS (and interacts with R31), are both translocated to the nucleus to differing degrees. Surprisingly after 30 min, the R31 K variant is present at high levels in the nucleus and at low levels in the cytoplasm, in neurites and on the cell membrane. After 120 min, it is still strongly in the nucleus. In comparison to R31K, the S28N variant at 30 min of uptake is present relatively weakly in the nucleus, cytoplasm and neurites and is absent on the cell membrane, the signal increases by 60 min and also appears on the cell membrane. At 120 min, the signal in the cytoplasm is relatively weak but the nuclear localization persists ( Fig. 2 ). The R31K ANG variant shows very little structural perturbation, which accounts for the negligible loss of RNase activity and the retention of nuclear translocation. On the other hand, the S28N ANG variant shows localized structural changes involving the NLS and this could explain the retardation in nuclear import. The seven variants in which the catalytic activity is affected—Q12L, K40I, I46V, P112L, V113I, H114R (all with attenuated RNase activity, some with very minimal activity) and R121H (with enhanced RNase activity)—exhibited different degrees of nuclear translocation ( Fig. 2 ). Low amounts of the P112L variant does get to the nucleus but most of the protein remains in the cytoplasm as large speckles and is absent from the neurites and membrane. At 120 min, the staining is mostly diffused in the cytoplasm. The most dramatic change in uptake and distribution is with the K17I and K17E variants. The nuclear translocation is minimal in K17I even at 120 min and at this time point the localization is mostly cytoplasmic and on the cell membrane. The substitution of Lys by Ile residue could indirectly affect the NLS region as they are in close proximity and this could account for the failure of this variant to translocate to the nucleus. The K17E is translocated in low amounts to the nucleus at 30 min with weak cytoplasmic staining. At 60 min, the staining is still weak, although at this time point there is faint staining in the neurites, by 120 min the staining in the nucleus and neurites is very strong with weak staining on the cell membrane ( Fig. 2 ). hANG-ALS variants affect MNs We have investigated the effects of the ANG-ALS variants on MNs derived from P19 EC cells. These ANG-ALS variant proteins have not been previously studied and exhibit a range of RNase activity (very low to high RNase activity). We assessed the effects of these variants on colony size, cell density, differentiation and survival of post-mitotic MNs. H114R and P112L are variants in the conserved region of the ANG molecule ( Fig. 1 ) and form a part of the catalytic apparatus with ~2% and 28% RNase activity, respectively, the K17I variant has 13% RNase activity and the R121H has significantly higher RNase activity (155%) compared with native hANG. P19 cells were induced to differentiate to neurons by co-culturing with the stromal cell line PA6 in the presence of retinoic acid (RA) for a period of 6 days. MNs were identified by staining for the MN markers—Islet 1 (ISL1 + ) and peripherin (Per + ). Using these conditions, we have previously shown that P19 cells induced to differentiate begin to form MNs on day 4 of differentiation and at day 6 of differentiation the colonies contain 10–12% post-mitotic MNs as seen by co-immunostaining for Peripherin (Per + ) and Islet 1 (ISL1 + ) [35] . In the current set of experiments, substantial sized neuronal colonies formed on the PA6 feeder layer on day 4 of differentiation in the untreated control cultures as seen by staining for neurofilament [35] . These colonies contain a proportion of cells that are both ISL1 + and Per + , which identifies them as post-mitotic MNs ( Supplementary Fig. S3 ). The Per + neurites within the colony form a mesh with stronger staining around the periphery. Per + dense cell bodies can be seen frequently at the periphery of the colonies and the Per + neurites of these neurons project out over the feeder layer. These neurites are relatively straight and are occasionally branched and make contact with the neurites from neighbouring colonies. ISL1 + nuclei within the colony also appear more frequently around the periphery of larger colonies and these neurites of these neurons express high levels of Per ( Supplementary Fig. S3 ). Per + -positive neurites present within colonies, and those projecting out over the PA6 increase in number and extent, through days 4, 5 and 6 of differentiation. This increase is also seen between days 4 and 6 in the presence of native ANG from day 4. However, the increase in the frequency of intensely Per + cells and accumulation at the edges of colonies is not as pronounced as in cultures treated with native ANG from day 0. Control cultures on day 5 of differentiation had a median of 8.2% (interquartile range (IQR) of 5.1–9.4%) ISL1 + nuclei within a colony and in cultures treated with native ANG this increased to 11.2% (IQR 5.1–15.7%) ISL1 + nuclei. The number of ISL1 + cells was significantly higher in cultures treated with native ANG ( P <0.05) when compared with cultures treated with: C39W (2.9% (IQR 1.2–5.1%)), H114R (2.8% (IQR 0.0–6.0)); K17I (1.9% (IQR 0.0–1.9%)), P112L (1.1% (IQR 0.0–4.3%)) and R121H (1.5% (IQR 0.0–3.6%)) variants. P19 cells differentiated to the neuronal lineage in the presence of native ANG from day 0 show much stronger Per + expression on day 5 ( Supplementary Fig. S4 ), as compared with those treated with the ANG-ALS variants. In the presence of WT ANG, there were more neurites at the periphery of the colonies than in the centre. ISL1 + nuclei were also seen more frequently at the edges of colonies than in its centre. The network of Per + neurites projecting from the colonies was similar to that in the control. On day 5 of differentiation, the neurites in the C39W variant treated cultures are thinner and stain weakly for peripherin ( Supplementary Fig. S4 i–l ) as compared with the untreated or WT treated cells. Fewer Per + neurites are present overall, and they rarely project out from the colonies. ISL1 + -positive cells are also rare within these colonies. Cells treated with the other ANG-ALS variants—K17I, H114R and P112L—also exhibited a similar phenotype ( Supplementary Fig. S4 m–p, q–t and u–y ) on day 5 of differentiation. In all of the ANG-ALS variant-treated cells, ISL1 + cells are present less frequently at the edges of the colony and additionally the Per + -positive neurites within a colony are very highly coiled and twisted. Neurites rarely project out from these colonies and those that extend out are highly curved. Overall, the numbers of Per + cells are substantially reduced on day 5 after treatment with the variant from day 0. In the case of cultures treated with R121H variant, the Per + neurites are considerably longer and stain more intensely for neurofilament but they too are highly coiled and rarely project out from the colony ( Supplementary Fig. S4z–ac ). Colonies treated with variants C39W and P112L from day 4 have reduced numbers of Per + -positive projections and Per + cell bodies ( Supplementary Fig. S5 i–l, u–x ). Where longer processes are present they frequently bend, kink or turn back on themselves. Small Per + swellings can frequently be seen in neurites projecting away from colonies ( Supplementary Fig. S5 . Filled arrowheads). Small numbers of Per + fragments are present on the PA6 cell layer. Fragmentation is seen more frequently in colonies treated with variants H114R, K17I and R121H from day 4 ( Supplementary Fig. S5 . Hollow arrowheads), as is the presence of kinked and clumped neurites. Comparison of frequency ISL1 + cells between colonies present after differentiation for 6 days without ANG variants and those treated from day 4 of differentiation shows that treatment with ANG variants H114R (2.1% (IQR 0.6–4.9%)), K17I (3.1% (IQR 2.0–5.3%)) and R121H (2.2% (IQR 0.8–5.7)) results in significantly lower numbers of ISL1 + cells ( P <0.05) on day 6. However, exposure to native ANG, variants C39W or P112L from day 4 did not result in a significant change in percentage of ISL1 + ( P <0.05; 12.9% (IQR 9.1–19.7%), 8.6% (IQR 4.8–13.6%) and 7.8% (IQR 4.4–12.2%), respectively). Differentiating cultures were treated with native hANG or hANG-ALS variants from day 0 of differentiation to assess their effects on differentiation and survival on days 5 and 6 after treatment. Six days after differentiation, the control cultures did not contain significantly different numbers of ISL1 + cells (10.6% (IQR 7.7–14.3%)) from those treated with native ANG from day 0 (12.7% (IQR 10.8–15.8%); Fig. 3a ). However, the control and native hANG-treated cultures both contain significantly higher numbers of ISL1 + cells ( P <0.05) than those treated from day 0 with: C39W (2.9% (IQR 1.2–5.1%)), H114R (2.8% (IQR 0.0–6.0%)), K17I (1.9% (IQR 0.0–1.9%)), P112L (1.1% (IQR 0.0–4.3%)) and R121H (1.5% (IQR 0.0–3.6%)) variants ( Fig. 3a ). Figure 3: Effects of WT hANG and hANG-ALS variants on post-mitotic motor neuron (MN) number and morphology. P19 cells were induced to differentiate to MNs by plating on PA6 feeder cells in the presence of RA as described in Supplementary Methods . Cells were differentiated in the presence or absence of hANG and hANG-ALS variant proteins from days 0 to 5 ( a ) and day 6 ( b ), or from days 4 to 6 only ( c ). Immunostaining for Islet 1 and Peripherin was used to determine the number of MNs per colony, whereas the total number of nuclei in a colony was found by DAPI staining, as described in Supplementary Information . Data were collected from two independent experiments ( n ≥10 colonies for each experiment). Median bars with interquartile range. Ball and arrow bars show where multiple conditions are significantly different from a single condition, whereas solid bars show significant differences between two conditions ( P 0.05, Log e transformed data compared by analysis of variance with Tukey's post hoc ). ( d ) Cells fixed on day 6 and stained for Peripherin (red) and Islet 1 (green) and counterstained with DAPI (blue). Cells were differentiated either in the absence of ANG (control) or in the presence of ANG WT, C39W, H114R, K17I, P112L or R121H variants. Filled arrows indicate kinked neurites. Hollow arrows indicate fragmented neurites. Scale bars, 50 μm. Full size image The neuronal colonies develop an extensive Per + neurite network expanding across the PA6 feeder layer in the absence of any ANG variants on day 6 of differentiation ( Fig. 3b ). A large proportion of cell bodies are intensely Per + and these cells are found frequently at the periphery of the colony. Neurites projecting from these colonies are relatively straight and curve infrequently. Again, Islet 1 is co-expressed in the nuclei of cells with Per + cell bodies, which also appear frequently at the edges of the colonies. Colonies are large with an extensive Per + -positive neurite network after six days of differentiation when treated with WT ANG ( Fig. 3b ). A large number of Per + -dense cell bodies are present throughout the colonies, mostly at the periphery accompanying extensive neurite projections away from the colony. These projections are very straight and rarely branched. ISL1 + nuclei are associated with highly Per + cell bodies, whereas a small number of ISL1 + Per − cells are present at the centres of some colonies. Peripherin is weakly expressed in the C39W variant-treated cultures ( Fig. 3b ). ISL1 + nuclei associated with Per + -dense cell bodies are present in fewer numbers and are frequently found in the centre of the colonies. These neurites often coil around the colony. Typically, very few Per + neurites project out from the colonies. A similar effect is also seen in cells treated with variants H114R, K17I and R121H ( Fig. 3b ). Considerable numbers of fragmented Per + neurites and neurites lacking a cell body are present in the H114R variant-treated cells. The cultures treated with the P112L variant form Per + networks of neurites similar to those in untreated or WT-treated cultures, but the ends of these neurites are highly branched and very frequently curved ( Fig. 3b ). Generally, neurites that extend from colonies treated with the ANG variants from day 0 are frequently kinked ( Fig. 3b , filled arrowheads) and fragmented ( Fig. 3b , hollow arrowheads). Effects of hANG-ALS variants on cell density and colony size Cell density in individual colonies was determined for each treatment and controls to assess the spread and migration of the neuronal cells when the cells were exposed to the variants on the day of induction of differentiation, that is, day 0. The cell density in untreated colonies (median of 248 DAPI + nuclei per colony (IQR 171–395)) on day 5 of differentiation is significantly higher ( P <0.05) than in colonies exposed to the ANG-ALS variants H114R (128 (IQR 80–175)), K17I (114 (IQR 69–169)) and R121H (131 (IQR 54–206); Supplementary Fig. S6 ). No significant differences were found between untreated colonies and those treated with native ANG (143 (IQR 100–265)), variants C39W (138 (IQR 80–209)) or P112L (133 (IQR 77–202); P <0.05). The cell density in colonies treated with native WT (median of 307 DAPI + nuclei per colony (IQR 205–368)) on day 6 is significantly higher ( P <0.05) than in colonies treated with variants K17I (141 (IQR 95–231)) and R121H (144 (IQR 117–268)) from day 0 ( Supplementary Fig. S6 ). No significant differences were found between the untreated colonies on day 6 (217 (IQR 142–324)) and native ANG, variants C39W (245 (IQR 137–353), H114R (203 (IQR 131–294)) or P112L (214 (IQR 122–292)). Similarly, no significant differences were found between the cell densities in control colonies on day 6 and those exposed to ANG variants when exposure to ANG and ANG-ALS variants was started on day 4 of differentiation ( Supplementary Fig. S6 ). Colony area was determined in cultures treated with hANG and ANG-ALS variants as well as controls for a period of 6 days from the initiation of differentiation on day 0. The areas of untreated colonies on day 5 of differentiation (21,542 μm 2 (IQR 13,807–27,529 μm 2 )) are significantly larger ( P <0.05) than those of colonies treated with either ANG variants K17I (9,140 μm 2 (IQR 4,971–14,854 μm 2 )) or P112L (8,873 μm 2 (IQR 4,718–16,243 μm 2 ); Supplementary Fig. S6 ). Colonies in cultures treated with native ANG (25,237 μm 2 (IQR 16,857–42,865 μm 2 )) were not significantly different from control untreated cultures. No significant differences were also observed in colony area between colonies in control untreated cultures ( P <0.05) and colonies in cultures treated with other ANG variants. The colony areas in control untreated cultures on day 6 (16,550 μm 2 (IQR 11,799–39,271 μm 2 )) are significantly larger ( P <0.05) than that of colonies in cultures treated with either K17I (9,765 μm 2 (IQR 7,150–16,589 μm 2 )) or R121H (8,934 μm 2 (IQR 5,658–20,068 μm 2 )) variants ( P <0.05). The area of the colonies in cultures treated with native ANG were also significantly larger than those treated with ANG variants H114R (14,990 μm 2 (IQR 10,297–19,202 μm 2 )), K17I and R121H ( P <0.05). Colonies treated with ANG variant C39W (20,845 μm 2 (IQR 12,373–29,776 μm 2 )) from day 0 also cover significantly larger areas than colonies treated with ANG variants K17I and R121H ( P <0.05; Supplementary Fig. S6 ). Treatment with hANG variants H114R (8,858 μm 2 (IQR 4,755–19,020 μm 2 )) or R121H (8,497 μm 2 (IQR 5,459–17,945 μm 2 )) for 48 h at day 4 of differentiation results in significantly reduced colony area when compared with untreated colonies ( Supplementary Fig. S6 ). No significant differences were found between areas of colonies in control cultures and colonies in cultures incubated with each of the other ANG variants. The areas of colonies treated with variant K17I (17,168 μm 2 (IQR 9,168–25,789 μm 2 )) from days 4 to 6 are significantly larger as compared with those in cultures treated from day 0 ( P <0.05). SY5Y cell lines expressing WT mAng1 haemagglutinin (HA) and ALS variants Mouse Ang1, the murine orthologue of hANG (with 76% amino-acid sequence identity) is expressed at high levels in neuronal cells including MNs [33] . We generated SY5Y neuronal cell lines stably expressing the WT mAng1 and two mAng1-ALS variants, which were epitope tagged (HA-tagged) using the constitutively active PN1 vector with the CMV promoter to assess the effect on survival, stress and TDP-43 distribution. The two ALS variants we chose were (a) K40I, which has a negligible RNase activity, and (b) C39W variant, which has reduced RNase activity and in which a disulphide bond is lost due to the mutation. Stable clones were isolated, genotyped ( Supplementary Fig. S7b ) and characterized for expression of the transgene by RT–PCR ( Supplementary Fig. S7c ), western blot and immunocytochemistry ( Supplementary Fig. S7d,e ). The morphology of the SY5Y mAng1 HA clone was similar to the untransfected SY5Y. The two mAng1 HA-ALS variant lines on the other hand were more aggregated. This was more pronounced in the SY5Y cells expressing K40I. ( Supplementary Fig. S7a ). Immunostaining with the anti-HA tag antibody revealed that the SY5Y mAng1 HA-transfected cells, the SY5Y mAng1 HA, K40I and the SY5Y mAng1 HA C39W cells expressed the HA-tagged proteins faintly in the nucleus and the cytoplasm but strongly in vesicles in the neurites ( Supplementary Fig. S7e ). Cell lysates from all three recombinant SY5Y cell lines contain a 17 kDa HA-tagged protein, which corresponds to the expected size of each mAng1HA with the signal sequence intact (16.2 kDa mAng1 plus 1.1 kDa HA tag) and which was absent in the lysates from the untransfected SY5Y. Each lysate also contains an additional band picked by the HA-tagged monoclonal antibody (mAb) around 21 kDa size ( Supplementary Fig. S7d ). Effects of stress on SY5Y cells expressing mAng1-ALS variants Stable SY5Y cells expressing HA epitope-tagged mAng1 (mAng1HA) and mAng1HA variants were used to study the effects on cell survival, responses to stress and cellular distribution of TDP-43. The untransfected SY5Y cells and the feeder PA6 are negative for the HA tag but stain positively for nuclear TDP-43. SY5Y cells normally express very low levels of neurofilament and have very short neurites. Untransfected and stably transfected SY5Y clones were differentiated to a more mature neuronal phenotype by co-culture with PA6 and RA treatment for a period of 6, 8 or 10 days. The differentiation to a mature neuronal phenotype was assessed by the increase in length of neurites and staining for neurofilament, which was maximal on day 10 of differentiation ( Fig. 4a–c ). We then analysed the effects on cell survival of the untransfected and transfected SY5Y clones at day 10. 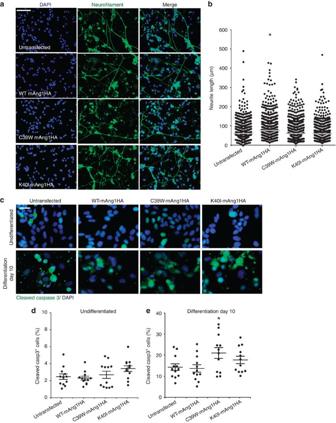Figure 4: Effect of mAng1-ALS variants on SY5Y neuronal morphology and survival. (a) Immunostaining for neurofilament expression in differentiated untransfected SY5Y and SY5Y cells expressing WT, C39W and K40I mAng1HA. SY5Y cells were differentiated by co-culturing with PA6 stromal cells in the presence of retinoic acid and dibutyryl-cAMP as described in Methods. Cells were immunostained for neurofilament expression using the 2H3 mAb (DSHB). Scale bar, 75 μm. (b) The lengths of neurofilament-positive neurites were measured in six randomly selected fields (660×490 μm2) from two independent experiments (median bars). Neurites of SY5Y cells expressing WT-mAng1HA are significantly longer than those of both untransfected SY5Y and SY5Y-expressing C39W or K40I mAng1HA (*P<0.05, SY5Yn=736, WTn=715, C39Wn=822, K40In=659, analysis of variance (ANOVA) with Tukey'spost hoc). (c) Immunostaining for cleaved caspase 3 in SY5Y clones both undifferentiated and differentiated on PA6 (with retinoic acid and dibutyryl-cAMP). (d) Undifferentiated cultures show no significant difference between the percentages of apoptotic cells present in each cell line. Scale bar, 25 μm. (e) Significantly more apoptotic SY5Y mAng1HA C39W cells (*P<0.05,n=6, ANOVA with Tukey'spost hoc) were found after differentiation when compared with untransfected SY5Y and SY5Y expressing WT or K40I mAng1HA. Cleaved caspase 3 and DAPI-positive cells were counted in six randomly selected fields (660×490 μm2) from two independent experiments. Fields of undifferentiated and differentiated cells contained an average of 480 cells (s.d.±198) and 415 cells (s.d.±252), respectively. Error bars±s.e.m. Figure 4: Effect of mAng1-ALS variants on SY5Y neuronal morphology and survival. ( a ) Immunostaining for neurofilament expression in differentiated untransfected SY5Y and SY5Y cells expressing WT, C39W and K40I mAng1HA. SY5Y cells were differentiated by co-culturing with PA6 stromal cells in the presence of retinoic acid and dibutyryl-cAMP as described in Methods. Cells were immunostained for neurofilament expression using the 2H3 mAb (DSHB). Scale bar, 75 μm. ( b ) The lengths of neurofilament-positive neurites were measured in six randomly selected fields (660×490 μm 2 ) from two independent experiments (median bars). Neurites of SY5Y cells expressing WT-mAng1HA are significantly longer than those of both untransfected SY5Y and SY5Y-expressing C39W or K40I mAng1HA (* P <0.05, SY5Y n =736, WT n =715, C39W n =822, K40I n =659, analysis of variance (ANOVA) with Tukey's post hoc ). ( c ) Immunostaining for cleaved caspase 3 in SY5Y clones both undifferentiated and differentiated on PA6 (with retinoic acid and dibutyryl-cAMP). ( d ) Undifferentiated cultures show no significant difference between the percentages of apoptotic cells present in each cell line. Scale bar, 25 μm. ( e ) Significantly more apoptotic SY5Y mAng1HA C39W cells (* P <0.05, n =6, ANOVA with Tukey's post hoc ) were found after differentiation when compared with untransfected SY5Y and SY5Y expressing WT or K40I mAng1HA. Cleaved caspase 3 and DAPI-positive cells were counted in six randomly selected fields (660×490 μm 2 ) from two independent experiments. Fields of undifferentiated and differentiated cells contained an average of 480 cells (s.d.±198) and 415 cells (s.d.±252), respectively. Error bars±s.e.m. Full size image The HA-tagged WT mAng1 appears as small punctate spots distributed throughout the cytoplasm with a weak nuclear signal ( Supplementary Fig. S7e ). The HA-positive vesicles appear evenly distributed throughout the soma and neurite of the cells with very strong staining at the tip of the neurite. In the mAng1HA C39W SY5Y cells, the staining for the mAng1 C39WHA is similar to that of the WT mAng1HA-expressing clone but a larger number of vesicles are seen in the soma rather than the distal tip of neurites. Branching of neurites appears to occur more frequently in shorter neurites compared with those of the WT-expressing clone. In the SY5Y mAng1HA K40I, the HA-positive punctate spots appear throughout the soma and neurites. They also appear more frequently in the soma than in WT-expressing clones and there is also some staining at the tip although relatively weak. The frequency of punctate spots in the soma does not appear to be as high as that seen in SY5Y mAng1HA C39W. The HA-positive punctate spots in the soma are larger than those seen in WT- or C39W-expressing cells and can also be seen in neurites. Expression of TDP-43 was nuclear in all four cell lines ( Supplementary Fig. S7e ). Apoptotic cells were present on day 10 of differentiation of SY5Y and mAng1-HA variant clones as seen by cells staining positive for cleaved caspase 3 with typically highly condensed or fragmented nuclei ( Fig. 4c ). No significant differences were found between the mean number of cells per field in which caspase 3 cleavage has occurred in undifferentiated SY5Y (2.5±1.1%) and SY5Y mAng1HA C39W (2.7±1.5%), K40I (3.4±1.2%) or WT (2.3±0.8%) cells. However, after ten days of differentiation many more SY5Y cells were positive for cleaved caspase 3 when compared with undifferentiated SY5Y. We found no significant differences in the numbers of cleaved caspase 3-positive cells between SY5Y (14.5±5.4%) and SY5Y mAng1HA K40I (17.9±6.1%) or SY5Y WT mAng1HA (13.9±6.1%) cells. However, there are significantly more cleaved caspase 3-positive cells in the SY5Y mAng1HA C39W (21.2±8.9%) cultures than in the untransfected SY5Y ( Fig. 4d,e ). A significantly higher percentage of differentiated SY5Y mAng1HA C39W cells were positive for cleaved caspase 3 as compared with the WT mAng1HA- and mAng1HA K40I-expressing clones. The viability of SY5Y cells is reduced when incubated with sodium arsenate at 0.5 or 1.0 mM but with no significant differences between the untransfected and the mAng1HA-expressing variants. Immunostaining showed redistribution of uniformly cytoplasmic eIF3η to distinct SGs to increasing degrees at 0.5 or 1.0 mM sodium arsenate. These SGs are frequently found adjacent to GE-1/hedls-positive processing bodies and extra-nuclear TDP-43 particularly at the higher concentration ( Fig. 5a ). Quantification of the SGs present in the cells indicates significant differences in response between untransfected SY5Y and the SY5Y cells expressing mAng1HA variants. The SY5Y clone expressing WT mAng1HA had significantly more SGs at 1.0 mM sodium arsenate (7.6 SG per cell ±0.57 s.e.m. ), whereas the K40I-expressing cells showed significantly fewer SGs (5.3 SG per cell ±0.32 s.e.m. ; P <0.05) than untransfected SY5Y cells (6.4 SG per cell ±0.61 s.e.m. ), while no significant effect is seen on SG induction in C39W-expressing cells (5.8 SG per cell ±073 s.e.m. ; Fig. 5b ). 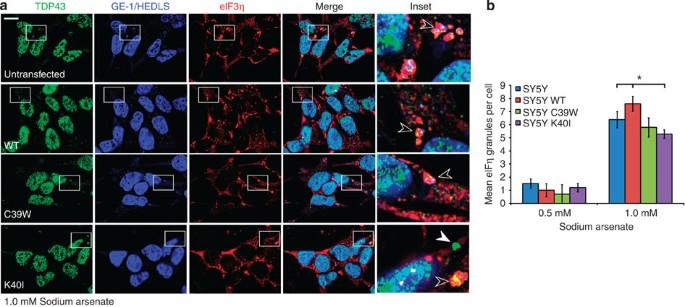Figure 5: Stress granule formation in SY5Y mAng1HA and mAng1HA-ALS cell lines. (a) Immunostaining for TDP-43, GE-1/HEDLS (processing bodies) and eIF3η (stress granules). SY5Y and SY5Y mAng1HA WT, C39W or K40I were treated with sodium arsenate for 2.5 h at the concentrations indicated. Open arrow indicates adjacent granules positive for all three markers, whereas closed arrow indicates single TDP-43 granules. Scale bar, 25 μm. (b) The number of eIF3η stress granules present in sodium arsenate-treated SY5Y (n=64), WT (n=62), C39W (n=78) or K40I (n=83). Data pooled from two experiments (*P<0.05): at 0.5 mM sodium arsenate SY5Y (n=51), WT (n=48), C39W (n=45), K40I (n=53) and at 1.0 mM sodium arsenate SY5Y (n=64), WT (n=62), C39W (n=78) and K40I (n=83). Analysis of variance with Tukey'spost hocanalysis). Error bars±s.e.m. Figure 5: Stress granule formation in SY5Y mAng1HA and mAng1HA-ALS cell lines. ( a ) Immunostaining for TDP-43, GE-1/HEDLS (processing bodies) and eIF3η (stress granules). SY5Y and SY5Y mAng1HA WT, C39W or K40I were treated with sodium arsenate for 2.5 h at the concentrations indicated. Open arrow indicates adjacent granules positive for all three markers, whereas closed arrow indicates single TDP-43 granules. Scale bar, 25 μm. ( b ) The number of eIF3η stress granules present in sodium arsenate-treated SY5Y ( n =64), WT ( n =62), C39W ( n =78) or K40I ( n =83). Data pooled from two experiments (* P <0.05): at 0.5 mM sodium arsenate SY5Y ( n =51), WT ( n =48), C39W ( n =45), K40I ( n =53) and at 1.0 mM sodium arsenate SY5Y ( n =64), WT ( n =62), C39W ( n =78) and K40I ( n =83). Analysis of variance with Tukey's post hoc analysis). Error bars±s.e.m. Full size image From our functional studies on the P19-derived MNs it is evident that the phenotypic effects of different mutations vary in their severity. One consistent finding is that all the ANG-ALS variants we have studied so far (the three reported in our previous study [34] ) and the four in the present study affect the survival of the MNs and neurite extension. It is also quite clear that the weak ribonucleolytic activity of ANG is a key to these processes. Both abrogation of the RNase activity and an increase in RNase activity have phenotypic consequences on the MNs. In the present study, the R121H variant, which has significantly higher RNase activity as compared with ANG, has very severe effects on the numbers of MNs, inhibits neurite extension leading to clumping of the neurites. It also causes neuronal degeneration as seen by the fragmented neurites. Several known members of the RNase A superfamily, such as onconase, amphinase, eosinophil-derived neurotoxin and eosinophil cationic protein, are cytotoxic and possess ribonucleolytic activity comparable to hANG-R121H variant. Variants Q12L, K40I, H114R, which are catalytically inactive, and the K17I variant, which has extremely low RNase activity, also have a very similar effect but with varying degrees of severity. It is interesting to note that the substitutions at the highly conserved K17 residue by Ile and Glu results in a significantly reduced RNase activity with diminished nuclear translocation concomitant with an increased toxicity towards neurons. It has been suggested that this residue forms part of the region involved in substrate binding and recognition of rRNA and is located close to the NLS. Structurally, the K17I variant shows significant changes and this might be responsible for its weak nuclear localization and increased toxicity. The K17E variant on the other hand has retained the full complement of van der Waals interactions, which would explain why its nuclear translocation is not as markedly affected. A suggested mechanism for ANG nuclear/nucleolar import involves passive diffusion of ANG through the nuclear pore and nucleolar-targeting signal-mediated nuclear/nucleolar retention, with cytoplasmic retention modulating the process [52] . Our uptake studies with the various hANG-ALS variants also support this possibility. In ANG-ALS variants, in which the NLS is perturbed structurally either due to a direct change in the NLS such as in R31K or indirectly through loss of interactions as in the case of S38N, P112L, K17I and K17E, the nuclear translocation occurs but to varying extents (not affected in R31K) and speed. It is likely that the modulation of the process of nuclear translocation is affected by the perturbations in the NLS. Therefore, it would seem that the overall conformation of NLS is more important than a single-residue change. What is clear is that the structural changes that lead to alterations in RNase activity of these variants are key to the phenotypic effects. The P112L mutant has very severe effects on the MN survival as well as in neurite extension although it retains 28% of the RNase activity of ANG. This could be explained by the fact that we (this study) and others observed that the translocation to the nucleus is affected [16] suggesting that besides the RNase activity, the nuclear translocation of ANG also is essential for some of its function. ANG has recently been shown to be important for SG assembly and the weak RNase activity is essential for this function [40] , [41] , [42] , [43] . The ability of ANG to induce the formation of SGs is likely to be important for MN survival and a loss of this function in the ANG-ALS variants is possibly responsible for the degeneration of the MNs carrying the ANG-ALS mutations. Stress granules have been identified in ALS spinal cord tissue. ALS mutants of the RNA metabolism proteins FUS [53] , [54] and TDP-43 (ref. 55 ) segregate into SGs and this increases when cells expressing these mutant proteins are subjected to stress. TDP-43 inclusions have been recently shown to be associated with SGs in both ALS and frontotemporal dementia [56] . In post-mortem brain, it has been shown to co-localize in inclusions containing TIA-1 (a cytotoxic granule-associated RNA-binding protein) and eukaryotic initiation factor 3 both of which are SG markers. We observed SG formation in SY5Y cells stably expressing the native mAng1 but not in the cells expressing the C39W/K40I ANG-ALS variants, suggesting that in neuronal cells the mechanisms of neuroprotection by ANG is mediated by its weak RNase activity through the SG pathway. The association of mutations in ANG and other proteins involved in RNA metabolism such as TDP-43 and FUS leading to altered stress responses and cell survival supports a role for this pathway in ALS and other neurodegenerative diseases and suggests a mechanism for the neuroprotective role of ANG. Expression and purification of native and ANG-ALS variants WT and all variants of ANG were prepared as reported in Holloway et al . [57] Briefly, a synthetic gene for WT ANG with Escherichia coli codon bias was inserted into pET-22b(+) (Novagen) for expression of the Met-(-1) form of the protein. The Stratagene QuikChange site-directed mutagenesis kit (Stratagene) was used to introduce mutations with the oligonucleotides listed as in Supplementary Information . After DNA sequencing (Cogenics, UK; MWG, Germany) to confirm the presence of the mutations, mutant plasmids were used to transform E. coli BL21(DE3) cells. Bacterial cells were grown in Terrific Broth at 37 °C to an OD 600 of 0.5–0.6, after which expression was induced by addition of isopropyl β- D -1-thiogalactopyranoside to a final concentration of 1 mM and incubation was continued for ~3 h before collecting. The target proteins from inclusion bodies were extracted, refolded and purified by SP-Sepharose chromatography followed by C4 reversed-phase HPLC [57] . Purified proteins were lyophilized and dissolved in AnalaR grade water. All ANG variants behaved similarly to the WT protein during purification. Concentrations of all recombinant proteins were determined from ultraviolet absorbance, using an 280 value of 12,500 M −1 cm −1 (ref. 58 ) calculated by the method described by Pace et al . [59] The purity of each protein was >98%, as judged by SDS–polyacrylamide gel electrophoresis and analytical scale reverse phase HPLC. The quality of the purified proteins was assessed by mass spectrometry, RNase assay and circular dichroism analysis (for details see Supplementary Information ). X-ray crystallographic studies Native ANG crystals were grown using hanging-drop vapour diffusion method in mother liquor 20% poly(ethylene glycol) (PEG) 4000, 0.05 M Na/K tartrate, 0.1 M NaCl, 0.1 M HEPES, pH 7.0 at 1:1 ratio. High-resolution X-ray diffraction data were recorded at 100 K, with PEG 4000 (30% (w/v)) as a cryoprotectant on a ADSC CCD Q315 detector at station I02 at Diamond Light Source, Oxon, UK. Three data sets at three different resolutions 1.8, 1.2 and 1.0 Å were collected, indexed, integrated and merged using HKL2000 software suite [60] to a high resolution of 1.04 Å resolution (for crystallographic statistics see Supplementary Table S1 ) in P2 1 2 1 2 (orthorhombic, with one molecule per asymmetric unit) space group. Initial phases were calculated by molecular replacement method using MOLREP software suite from CCP4 package [61] and native ANG (PDB ID: 1ANG [30] ) as the starting model. Subsequent model building and X-ray structural refinement (anisotropic) was carried out using COOT [62] and PHENIX software package [63] , respectively. A set of 5% of randomly selected reflections was kept aside for use in R free calculation. Visible bound water and tartrate molecules were modelled into the electron density using difference density map (Fo-Fc) after all the protein atoms were built. Several amino-acid residues were found to have more than one conformation, and these alternate conformations were modelled, refined and built into the final structure. The residues in alternate conformations are Thr7, Pro18, Gln19, Gly20, Arg21, Ser28, Arg31, Ser37, Lys40, Asp41, Ser52, Pro64, Ser72, Lys73, Thr97 and Ala98. The structure was refined to a final R cryst and R free value of 0.169 and 0.188, respectively, with 2 tartrate and 159 water molecules. There were 97.5% of residues in most favourable region of Ramachandran plot with 2.5% in the generously allowed region ( Supplementary Table S1 ). Variant ANG proteins were crystallized using the hanging-drop method (for detailed conditions used see Supplementary Table S1 ). Diffraction data for all the ANG-ALS variants were collected at 100 K, with PEG 4000 (30%, w/v) or 25 % glycerol as a cryoprotectant, on stations PX 10.1 and 14.2 at the Synchrotron Radiation Source (Daresbury, UK) using a Quantum-4 CCD detector (ADSC Systems, Poway, CA, USA), Diamond Light Source (stations I02 and I04) using a Quantum-4 CCD detector and the in-house X-ray source Rigaku Micromax 007 HF. Data were processed and scaled using HKL2000 software suite [60] . Initial phases were obtained by molecular replacement method using 1ANG as the starting model [30] . Further refinement and model building were carried out with PHENIX [63] and COOT [62] , respectively ( Supplementary Table S1 ). With each data set, a set of reflections (5%) was kept aside for the calculation of R free . All the structures were validated using MolProbity validation tool [64] . There were no residues in the disallowed region of the Ramachandran plot. Crystallographic data statistics are summarized in Supplementary Table S1 . All figures were drawn with PyMOL (DeLano Scientific LLC, San Carlos, CA, USA) and rendered with POV-ray. Hydrogen bonds were verified with the programme HBPLUS. Molecular modelling studies In the case of C39W [5] , T80S [8] , F100I [8] , V103I [7] , H114R [14] and R121C [9] variants (where the crystal structures are yet to be determined), ALS mutations were modelled using the atomic resolution crystal structure of ANG. Individual mutations were introduced into the structure using the graphics programme COOT [62] . All the mutated models were then subjected to 200 steps of conjugate gradient minimization using the programme CNS [65] . This was followed by an annealing schedule with a starting molecular dynamics temperature of 298 K. Cloning of mAng1HA and ALS variant expression constructs The coding sequence of mAng1 including the signal peptide was amplified by PCR from mouse genomic DNA. This was used as a template for generating the coding sequence with the HA tag at the C-terminal end and cloned into Bluescript and verified by sequencing. The ALS mutations were introduced by site-directed mutagenesis using the Stratagene site-directed mutagenesis kit. The WT and Ang ALS variant sequences were then cloned into PN1 (Clontech) vector from which the green fluorescent protein had been removed. All expression constructs were authenticated by sequencing. Cell culture and transfections Mouse embryonal carcinoma cells P19 (ref. 66 ) and PA6 stromal cells [67] were grown in alpha minimum essential medium with glutamax (alpha-MEM, Invitrogen) supplemented with 10% FCS (Invitrogen) and 1% non essential amino acids (NEAA, Invitrogen) at 37 °C in 5% CO 2 . SY5Y cells were routinely cultured in DMEM:F12 with glutamax (Invitrogen) supplemented with 1% NEAA (Invitrogen) and 10% FCS. SY5Y cells were transfected with expression constructs using Fugene 6 (Roche) following manufacturer's instructions and colonies resistant to G418 were isolated and expanded. Stable transfectants were confirmed by PCR using ANG forward and HA reverse primers. SY5Y differentiation Subconfluent PA6 stromal cells were plated on gelatinzed glass coverslips in 24-well plates in alpha-MEM with glutamax and 15% FCS and allowed to grow to confleuncy (by 48 h). SY5Y were seeded on the PA6 feeder layer at a density of 5,000 cells per well in 0.5 ml differentiation medium (DMEM:F12 with glutamax (Invitrogen), 1% NEAA (Invitrogen), 0.5% KOSR (Invitrogen) and 10 μM All RA (Sigma)). Differentiation medium was changed every 48 h. Uptake of hANG and hANG-ALS variants by SY5Y cells Subconfluent SY5Y (~70%) grown on glass coverslips in 24-well plates were incubated for 30–120 min in culture medium containing 200 ng ml −1 of hANG and ANG-ALS variants. The cells were fixed in cold methanol/acetic acid (3:1) for 20 min. The coverslip cultures were rehydrated and stained for hANG with the 26-2F mAb and Alexa 488-conjugated anti-mouse secondary antibody. Z-stacked Images were acquired using a Leica DFC6000 camera (Leica) and DM55 microscope and deconvoluted using the LAS software. Immunocytochemistry Cells were fixed in 4% paraformaldehyde in PBS or in ice-cold methanol and washed with PBS, nonspecific binding was blocked in blocking buffer (PBS with 0.1%. gelatin, 0.5% BSA and 0.1% Tween-20) for 1 h at room temperature. The primary antibodies used for staining MNs were mouse anti-Islet 1 (1:5, 40.2D6 DSHB), rabbit anti-peripherin (Chemicon) and anti-neurofilament antibody (1:5, 2H3, DSHB). Expression of the transgene in transfected cells was confirmed by immunostaining using the HA.11 anti-HA monoclonal antibody from Covance. Immunostaining for other antigens was performed using Rabbit Anti-TDP-43 (1:1,000, Proteintech group), Mouse Anti-hedls (1:1,000, SantaCruz) and Goat Anti-eiF3η (1:200, SantaCruz). Primary antibodies diluted in block buffer were allowed to bind overnight at 4 °C with shaking, washed with 0.1% (v/v) of Triton X-100 in PBS (3×10 min). The cells were incubated with appropriate secondary antibody for 1 h at room temperature. Secondary antibodies were goat anti-mouse Alexa 488 (1:1,000, Molecular probes) and goat anti-mouse Alexa 594 (1:1,000, Molecular probes), AlexaFluor 350 donkey anti-mouse IgG (H+L) and AlexaFluor 594 donkey anti-goat IgG (H+L) (1:2,000, Invitrogen). Cells were washed with wash buffer and stained with 4',6-diamidino-2-phenylindole (DAPI; 0.1 μg ml −1 , Sigma) in PBS for 5 min at room temperature and mounted in Mowiol. Staining was observed using a Leica DM55 microscope and images captured using a DFC-6000 camera and processed using LAS software. Stress granule assay SY5Y cells stably expressing WT mAng1HA, mAng1ALS K40I HA and mAng1ALS C39WHA were plated on coverslips in 24-well plates and treated with sodium arsenate at 0.5 and 1.0 mM as described by Ivanov et al . [68] Cells were fixed in 4% PFA and stained for SG marker eIF3η, hedls and for TDP-43. Number of SGs were counted for all the cell lines and compared with untransfected SY5Y. Images were acquired using a Leica DM55 and analysed using the Leica LAS programme. Z-stacked images were acquired using a Leica DM55 microscope and deconvoluted using the LAS software. Data from two independent experiments were pooled and compared by analysis of variance with Tukey's post-hoc test. Additional details of the experimental methods used in this study are available under Supplementary Information . Accession codes: The atomic coordinates and structure factor amplitudes have been deposited with the Protein Data Bank ( http://www.pdb.org ; PDB ID codes are— 4AOH for hANG atomic resolution structure; 4AHD , 4AHE , 4AHF , 4AHG , 4AHH , 4AHI , 4AHJ , 4AHK , 4AHL , 4AHM , 4AHN for Q12L , K17E , K17I , S28N , R31K , K40I , I46V , K54E , P112L , V113I , R121H for hANG-ALS variants, respectively). How to cite this article: Thiyagarajan N. et al . Structural and molecular insights into the mechanism of action of human angiogenin-ALS variants in neurons. Nat. Commun. 3:1121 doi: 10.1038/2126 (2012).